Knockdown and knockout of β1-integrin in hepatocytes impairs liver regeneration through inhibition of growth factor signalling The liver has a unique regenerative capability, which involves extensive remodelling of cell–cell and cell–matrix contacts. Here we study the role of integrins in mouse liver regeneration using Cre/loxP-mediated gene deletion or intravenous delivery of β1-integrin siRNA formulated into nanoparticles that predominantly target hepatocytes. We show that although short-term loss of β1-integrin has no obvious consequences for normal livers, partial hepatectomy leads to severe liver necrosis and reduced hepatocyte proliferation. Mechanistically, loss of β1-integrin in hepatocytes impairs ligand-induced phosphorylation of the epidermal growth factor and hepatocyte growth factor receptors, thereby attenuating downstream receptor signalling in vitro and in vivo . These results identify a crucial role and novel mechanism of action of β1-integrins in liver regeneration and demonstrate that protein depletion by nanoparticle-based delivery of specific siRNA is a powerful strategy to study gene function in the regenerating liver. Because of the essential functions of the liver in metabolism and compound detoxification, it is pivotal to guarantee a rapid and efficient repair of the organ after injury caused by viruses, toxins or autoimmune attacks, as well as after liver transplantation or tumour surgery. The model of two-third partial hepatectomy (PH) in rodents is widely used to study the different stages of liver regeneration, including hepatocyte cell cycle entry, cell proliferation and termination, which finally result in the restoration of the initial liver mass [1] , [2] . Growth factors, cytokines and their corresponding receptors control these different stages, and regulate activation, proliferation and survival of liver cells during the regeneration process [3] . Although hepatocytes express multiple adhesion molecules, including integrins, surprisingly little is known about their roles in liver regeneration. Integrins form a large family of transmembrane cell surface receptors, comprising 18 α- and 8 β-subunits that assemble into 24 non-covalently associated heterodimers with distinct, but overlapping specificities for ligands [4] . Besides their role in cell anchorage via cell–cell and cell–matrix interactions, integrins assemble large signalling hubs that control cell survival, proliferation, differentiation and migration in normal, injured and cancerous tissues [4] , [5] , [6] . The β1-integrin subunit (Itgb1) associates with at least ten α-subunits, giving rise to the largest integrin subfamily [4] . Interestingly, gene expression profiling revealed that various genes involved in the integrin signalling pathway were regulated during rat liver regeneration [7] . This is obviously of functional relevance, as liver-specific ablation of integrin-linked kinase (ILK) interfered with the proper termination of liver regeneration, resulting in enlarged livers after PH [8] . However, the role of individual integrin subunits in liver regeneration has not been determined and their mechanisms of action in the normal and regenerating liver remain to be investigated. In this study we used a dual approach to study the role of Itgb1 in liver regeneration—inducible Cre/loxP-mediated gene deletion and small interfering RNA (siRNA)-mediated knockdown in hepatocytes in vivo . The use of genetically modified mice with gain- or loss-of-function of individual genes is the gold standard to study the involvement of proteins in a biological process in vivo . Their use for liver regeneration studies identified the contribution of growth factors and their corresponding receptors to this process. Of particular importance are the hepatocyte growth factor (HGF) receptor c-Met and the epidermal growth factor receptor (EGFR). Inducible deletion of c-Met in the liver resulted in reduced hepatocyte proliferation and concomitant impairment of liver regeneration [9] . Constitutive hepatocyte-specific knockout of c-Met caused severe liver necrosis after PH and reduced the survival of the animals [10] . Mice lacking the EGFR in the liver showed increased mortality, liver cell damage and reduced hepatocye proliferation, resulting from a defective entry into the G1–S phase of the cell cycle [11] . Considerable effort has been directed towards developing effective delivery systems for siRNAs in vivo [12] , [13] , [14] . Plasmid-based expression of short hairpin RNA has been used to study the role(s) of HGF/c-Met and EGFR during liver regeneration in rats [15] , [16] , and stable delivery of pools of short hairpin RNAs into mouse livers lead to the identification of the kinase MKK4 as a major regulator of liver regeneration [17] . Additional siRNA delivery systems were invented to improve tissue specificity and low-dose efficacy. In particular, lipid nanoparticle formulations were developed, which efficiently and predominantly delivered siRNA to the liver and allowed knockdown of several genes simultaneously after a single injection of multiple siRNAs [18] , [19] , [20] . Therefore, we used this powerful strategy in combination with a knockout approach to determine the outcome of the loss of β1-integrin in hepatocytes for liver regeneration after PH. In a parallel study, Bogorad et al. [21] studied the role of β1-integrin in hepatocytes for liver homeostasis and carcinogenesis. Here we demonstrate an important role of β1-integrins in liver regeneration through regulation of signalling by major growth factor receptors. In addition, we show that nanoparticle-based delivery of siRNA is a powerful strategy to study gene function in the regenerating liver. Generation of mice lacking Itgb1 in the liver Mice with floxed Itgb1 alleles (Itgb1 f/f mice) [22] were mated with MxCre mice, in which Cre expression can be induced by injection of poly-IC. This has been shown to result in complete deletion of floxed alleles in the liver and to almost complete deletion in the spleen. By contrast, deletion in other tissues is much less efficient or even absent [23] . The double transgenic progeny was designated Itgb1 f/f /MxCre mice [24] , [25] . Mice were injected twice with a 2-day interval with poly-IC. Already 14 days after the last poly-IC injection, the Itgb1 alleles were efficiently deleted in the liver of Itgb1 f/f /MxCre mice as shown by staining for β-galactosidase (β-gal), whose expression is induced on deletion of the floxed allele [22] ( Fig. 1a ). No staining was seen in the intestine where recombination had not occurred ( Fig. 1b ). As expected, a strong reduction in the levels of Itgb1 mRNA was also seen in the spleen, although to a much lesser extent than in the liver. No reduction was seen in the lung ( Fig. 1c ). Immunofluorescence staining verified the efficient gene knockout in hepatocytes ( Fig. 1d ), whereas platelet/endothelial cell adhesion molecule 1 (PECAM-1)-positive endothelial cells were still Itgb1 positive ( Fig. 2a ). In addition, co-staining for Itgb1 and F4/80 or α-smooth muscle actin (α-SMA) showed that Kupffer cells and activated hepatic stellate cells/myofibroblasts also remained Itgb1 positive ( Fig. 2b,c ). Therefore, Mx-Cre-mediated loss of Itgb1 was obviously restricted to hepatocytes, whereas deletion in other cells of the liver was inefficient. Poly-IC-injected Itgb1 f/f /MxCre mice did not show obvious health impairments, and a histological analysis of liver tissue showed no gross morphological abnormalities during the first 4 weeks after Itgb1 deletion ( Supplementary Fig. 1A ). Furthermore, there were no obvious vascular abnormalities as shown by PECAM-1 staining ( Supplementary Fig. 1B ). However, despite the normal liver morphology, serum activities of aspartate aminotransferase, alanine aminotransferase and lactate dehydrogenase, and serum concentrations of bilirubin were increased 14 days after poly-IC injection, indicating initiation of liver damage by knockout of Itgb1 ( Supplementary Fig. 1C ). By contrast, albumin levels were not affected, suggesting that liver function is not severely compromised ( Supplementary Fig. 1C ). In line with these findings, all animals survived the observation period. 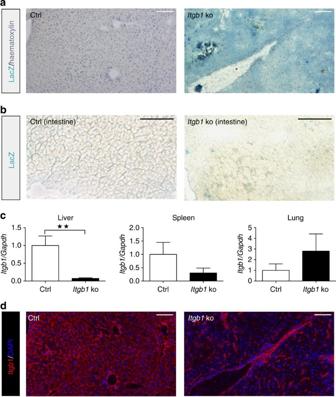Figure 1: Mx-Cre-mediated knockout ofItgb1occurs predominantly in hepatocytes. Cre-mediated deletion of theItgb1alleles, resulting in knockout ofItgb1and concomitant expression of β-galactosidase, was analysed by lacZ staining on sections from the liver (a) and intestine (b), from poly-IC-treatedItgb1f/f/MxCremice (Itgb1 ko) and control littermates (ctrl). (c)Itgb1mRNA levels relative toGapdhwere analysed by qRT–PCR using RNAs from the liver, spleen and lung. Bars represent mean±s.e.m.N≥3 per genotype. **P≤0.01 (Mann–WhitneyU-test). (d) Immunofluorescence staining for Itgb1 (red) was performed on liver sections fromItgb1f/f/MxCremice (Itgb1 ko) and control littermates (ctrl). Nuclei were counterstained with DAPI (blue). Scale bars, 100 μm (a–d). Figure 1: Mx-Cre-mediated knockout of Itgb1 occurs predominantly in hepatocytes. Cre-mediated deletion of the Itgb1 alleles, resulting in knockout of Itgb1 and concomitant expression of β-galactosidase, was analysed by lacZ staining on sections from the liver ( a ) and intestine ( b ), from poly-IC-treated Itgb1 f/f /MxCre mice (Itgb1 ko) and control littermates (ctrl). ( c ) Itgb1 mRNA levels relative to Gapdh were analysed by qRT–PCR using RNAs from the liver, spleen and lung. Bars represent mean±s.e.m. N ≥3 per genotype. ** P ≤0.01 (Mann–Whitney U -test). ( d ) Immunofluorescence staining for Itgb1 (red) was performed on liver sections from Itgb1 f/f /MxCre mice (Itgb1 ko) and control littermates (ctrl). Nuclei were counterstained with DAPI (blue). Scale bars, 100 μm ( a – d ). 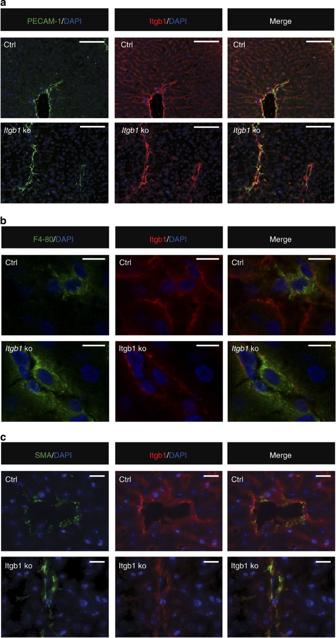Figure 2: Hepatic non-parenchmal cells retain Itgb1 expression after Mx-Cre-mediated Itgb1 deletion. Co-staining for Itgb1 (red) and PECAM-1 (green) (a) or F4/80 (green) (b), or α-smooth muscle actin (SMA) (green) of liver sections from poly-IC-treated Itgb1f/f/MxCre and MxCre control mice. Nuclei were stained with DAPI (blue). (N≥3). Representative pictures were chosen. Scale bars, 100 μm (a) and 20 μm (b,c). Full size image Figure 2: Hepatic non-parenchmal cells retain Itgb1 expression after Mx-Cre-mediated Itgb1 deletion. Co-staining for Itgb1 (red) and PECAM-1 (green) ( a ) or F4/80 (green) ( b ), or α-smooth muscle actin (SMA) (green) of liver sections from poly-IC-treated Itgb1 f/f /MxCre and MxCre control mice. Nuclei were stained with DAPI (blue). ( N ≥3). Representative pictures were chosen. Scale bars, 100 μm ( a ) and 20 μm ( b , c ). Full size image Itgb1 is required for liver regeneration after PH Fourteen days after the second poly-IC injection, mice were subjected to PH. Our complete treatment scheme, shown schematically in Fig. 3a , caused 47% lethality of Itgb1 f/f /MxCre mice, but only 7% lethality in control mice within 24–48 h after PH ( Fig. 3b ). As all Itgb1 f/f /MxCre mice survived the first 24 h after surgery, we conclude that a defect in the onset of regeneration and/or metabolic abnormalities rather than acute surgical complications caused the death of the animals. 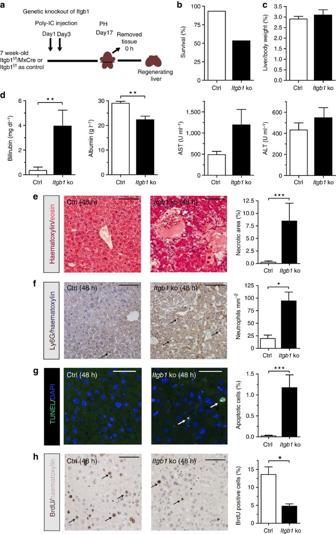Figure 3: Loss of Itgb1 causes severe defects in liver regeneration after PH. (a) Scheme of poly-IC-induced knockout ofItgb1. (b) Survival index 48 h after PH.N≥16 mice per genotype. (c) Liver-to-body-weight ratio 48 h after PH. (d) Aspartate aminotransferase (AST) and alanine aminotransferase (ALT) activities, bilirubin and albumin levels in the serum 48 h after PH of control (white bars) and Itgb1f/f/MxCre mice (black bars).N≥8 per genotype. (e) Representative pictures of liver tissue and quantification of necrotic area.N≥10 per genotype. (f) immunostaining for neutrophils and quantification.N≥3.; Ly-6G-positive cells are indicated by arrows, (g) TUNEL staining of apoptotic cells and quantification.N≥7; TUNEL-positive nuclei are indicated by arrows. (h) BrdU immunostaining and quantification 48 h after PH of poly-IC-treated control (white bars) and Itgb1f/f/MxCre mice (black bars.N≥5. BrdU-positive nuclei are indicated by arrows. Scale bars, 100 μm. Bars inb–hrepresent mean±s.e.m. *P≤0.05, **P≤0.01 and ***P≤0.001 (Mann–WhitneyU-test). Figure 3: Loss of Itgb1 causes severe defects in liver regeneration after PH. ( a ) Scheme of poly-IC-induced knockout of Itgb1 . ( b ) Survival index 48 h after PH. N ≥16 mice per genotype. ( c ) Liver-to-body-weight ratio 48 h after PH. ( d ) Aspartate aminotransferase (AST) and alanine aminotransferase (ALT) activities, bilirubin and albumin levels in the serum 48 h after PH of control (white bars) and Itgb1 f/f /MxCre mice (black bars). N ≥8 per genotype. ( e ) Representative pictures of liver tissue and quantification of necrotic area. N ≥10 per genotype. ( f ) immunostaining for neutrophils and quantification. N ≥3. ; Ly-6G-positive cells are indicated by arrows, ( g ) TUNEL staining of apoptotic cells and quantification. N ≥7; TUNEL-positive nuclei are indicated by arrows. ( h ) BrdU immunostaining and quantification 48 h after PH of poly-IC-treated control (white bars) and Itgb1 f/f /MxCre mice (black bars. N ≥5. BrdU-positive nuclei are indicated by arrows. Scale bars, 100 μm. Bars in b – h represent mean±s.e.m. * P ≤0.05, ** P ≤0.01 and *** P ≤0.001 (Mann–Whitney U -test). Full size image The liver-to-body-weight ratio was not significantly different between Itgb1 f/f /MxCre and control mice at 48 h after surgery ( Fig. 3c ). However, we detected a further increase in the activities of alanine aminotransferase, aspartate aminotransferase and lactate dehydrogenase, enhanced levels of bilirubin and reduced levels of albumin in the serum of Itgb1 f/f /MxCre mice 48 h after PH, indicating liver damage and impaired liver function ( Fig. 3d ). Indeed, Itgb1 f/f /MxCre mice displayed severe liver necrosis 48 h after PH ( Fig. 3e ), which was accompanied by enhanced infiltration of neutrophils ( Fig. 3f ). The number of apoptotic cells as determined by TUNEL (TdT-mediated dUTP nick end labelling) staining ( Fig. 3g ) or staining for cleaved caspase-3 ( Supplementary Fig. 1D ) was also increased, while the hyperproliferation of hepatocytes that occurred in control mice 48 h after PH was strongly reduced in Itgb1 f/f /MxCre mice ( Fig. 3h ). As poly-IC-induced expression of Cre recombinase also occurs in haematopoietic cells, we generated bone marrow chimeric mice by transplanting Itgb1 f/f /MxCre bone marrow into γ-irradiated wild-type mice, and we subsequently induced Itgb1 deletion in blood cells. Successful transfer of the bone marrow and poly-IC-induced knockout after complete engraftment of the recipient mice was verified by the detection of β-gal activity in platelets of bone marrow chimeric mice ( Fig. 4a ). None of the animals showed tissue damage 48 h after PH ( Fig. 4b ), indicating that loss of Itgb1 in haematopoietic cells is not the primary reason for the regeneration defect of poly-IC-treated Itgb1 f/f /MxCre mice. Rather, the regeneration defect in Itgb1 f/f /MxCre mice results from loss of Itgb1 in hepatocytes. 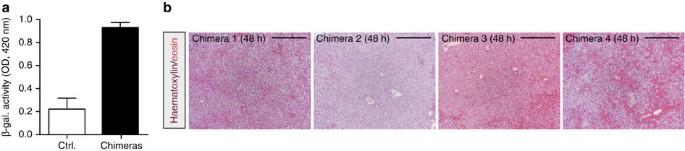Figure 4: Loss ofItgb1in immune cells does not impair liver regeneration after PH. Bone marrow chimeric mice were generated by transfer of bone marrow from Itgb1f/f/MxCre mice into lethally irradiated control mice. (a) Two weeks after the first injection of poly-IC, β-gal activity was analysed in platelet lysates from chimeric and control mice.N≥3. Bars indicate mean±s.e.m. (b) Liver sections from four different bone marrow chimeric mice that had been treated with poly-IC were analysed by haematoxylin/eosin staining. Note the lack of necrosis. Scale bar, 500 μm. Figure 4: Loss of Itgb1 in immune cells does not impair liver regeneration after PH. Bone marrow chimeric mice were generated by transfer of bone marrow from Itgb1 f/f /MxCre mice into lethally irradiated control mice. ( a ) Two weeks after the first injection of poly-IC, β-gal activity was analysed in platelet lysates from chimeric and control mice. N ≥3. Bars indicate mean±s.e.m. ( b ) Liver sections from four different bone marrow chimeric mice that had been treated with poly-IC were analysed by haematoxylin/eosin staining. Note the lack of necrosis. Scale bar, 500 μm. Full size image Knockdown of Itgb1 in hepatocytes in vivo To verify the importance of Itgb1 in hepatocytes for liver regeneration after PH and to compare the outcome after genetic knockout with siRNA-mediated knockdown in hepatocytes in vivo , we used lipid-based nanoparticles to deliver Itgb1 siRNA, which had been optimized for liver-specific targeting and which preferentially target hepatocytes [19] . A single injection of Itgb1 siRNA reduced Itgb1 mRNA levels by >85% in comparison with an injection with luciferase (Luc) siRNA, which was used as a negative control. Importantly, the knockdown was maintained for more than 10 days after a single injection of siRNA [21] . As a consequence of the Itgb1 knockdown, adhesion of isolated hepatoctytes on collagen was strongly reduced [21] . To ensure a prolonged and efficient knockdown as a pre-requisite to study the role of Itgb1 in liver regeneration, we injected siRNA twice within a 5-day interval. Five days after the last injection, the animals were subjected to PH as shown schematically in Fig. 5a . At the time of surgery, the liver tissue showed a >90% reduction in Itgb1 mRNA levels ( Fig. 5b ). Western blotting revealed an siRNA-mediated reduction of Itgb1 protein in total liver lysates, and a complete loss of Itgb1 protein in purified primary hepatocytes, indicating that the residual Itgb1 detected in total liver results from expression in non-parenchymal liver cells, which were apparently not efficiently targeted by the nanoparticles ( Fig. 5c ). Itgb1 immunostaining of the tissue removed during surgery and 48 h after PH confirmed the knockdown in hepatocytes ( Fig. 5d ), while co-staining of Itgb1 with PECAM-1, α-SMA or F4/80 revealed that endothelial cells, activated stellate cells/myofibroblasts and Kupffer cells were still Itgb1 positive ( Fig. 5e–g ). 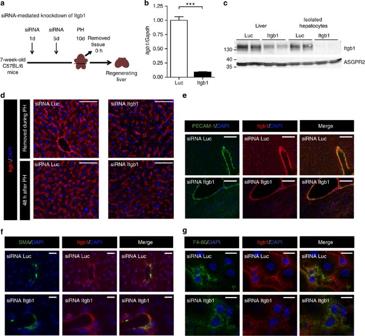Figure 5: Efficient hepatocyte-specific knockdown ofItgb1 in vivo. (a) Scheme of siRNA-mediatedItgb1knockdown and the following PH experiment. Mice were treated twice with siRNA against luciferase(Luc) or Itgb1 (Itgb1) with a time interval of 5 days. After additional 5 days, animals were used for experiments. (b) Verification of siRNA-mediated knockdown ofItgb1mRNA in the liver by qRT–PCR (normalized toGapdh) 5 days after the second siRNA injection. Scale bars indicate mean±s.e.m;N≥8 per treatment group. ***P≤0.001 (Mann–WhitneyU-test). (c) Immunoblotting of Itgb1 and asialoglycoprotein receptor (ASGPR2) as loading control using total liver homogenates or lysates from isolated primary hepatocytes after siRNA-mediated knockdownin vivo. (d) Immunostaining for Itgb1 (red) and DAPI nuclear counterstain (blue) on cryosections of tissue removed during PH and 48 h after PH. (e–g) Co-staining was performed for Itgb1 (red) and PECAM-1 (green,e), α-smooth muscle actin (SMA) (green,f) or F4/80 (green,g) on liver tissue slides 5 days after the secondItgb1or luciferase siRNA injection. Nuclei were stained with DAPI (blue).N≥3. Representative pictures were chosen. Scale bars, 100 μm (d,e) and 20 μm in (f,g). Figure 5: Efficient hepatocyte-specific knockdown of Itgb1 in vivo . ( a ) Scheme of siRNA-mediated Itgb1 knockdown and the following PH experiment. Mice were treated twice with siRNA against luciferas e ( Luc ) or Itgb1 ( Itgb1 ) with a time interval of 5 days. After additional 5 days, animals were used for experiments. ( b ) Verification of siRNA-mediated knockdown of Itgb1 mRNA in the liver by qRT–PCR (normalized to Gapdh ) 5 days after the second siRNA injection. Scale bars indicate mean±s.e.m; N ≥8 per treatment group. *** P ≤0.001 (Mann–Whitney U -test). ( c ) Immunoblotting of Itgb1 and asialoglycoprotein receptor (ASGPR2) as loading control using total liver homogenates or lysates from isolated primary hepatocytes after siRNA-mediated knockdown in vivo . ( d ) Immunostaining for Itgb1 (red) and DAPI nuclear counterstain (blue) on cryosections of tissue removed during PH and 48 h after PH. ( e – g ) Co-staining was performed for Itgb1 (red) and PECAM-1 (green, e ), α-smooth muscle actin (SMA) (green, f ) or F4/80 (green, g ) on liver tissue slides 5 days after the second Itgb1 or luciferase siRNA injection. Nuclei were stained with DAPI (blue). N ≥3. Representative pictures were chosen. Scale bars, 100 μm ( d , e ) and 20 μm in ( f , g ). Full size image Consistent with previous findings demonstrating that >90% of injected siRNA-loaded lipid nanoparticles accumulated in the liver [26] , no reduction in the mRNA levels of Itgb1 was observed in the lung, kidney and heart ( Supplementary Fig. 2A ), or in the blood, bone marrow or brain [21] . Spleen was the only tissue in which siRNA-loaded nanoparticles reduced Itgb1 mRNA levels by ~\n50% ( Supplementary Fig. 2A ). We assume that the Itgb1 reduction in spleen is unlikely causing phenotypic abnormalities, as a constitutive heterozygous deletion of the Itgb1 gene in mice lead to no apparent defects [27] , and as the loss of Itgb1 in haematopoietic cells did not affect the normal liver or the regeneration process after PH (see above). The siRNA treatment neither induced the expression of interferon-γ mRNA under our experimental conditions, nor histological or vascular abnormalities in the liver at day 5 after the second siRNA injection ( Supplementary Fig. 2B,C ). In contrast to the knockout mice, serum parameters remained normal on Itgb1 knockdown ( Supplementary Fig. 2D ) and all animals survived the observation period. Itgb1 knockdown leads to a mild regeneration defect In contrast to Itgb1 f/f /MxCre mice, the survival of Itgb1 knockdown animals was not reduced 48 h after PH ( Fig. 6a ). Surprisingly, the animals even showed an increase in liver-to-body-weight ratio compared with control animals ( Fig. 6b ). At the histological level, however, we found similar abnormalities in Itgb1 knockdown and knockout animals, including severe necrotic tissue damage, concomitant neutrophil infiltration ( Fig. 6c,d ) and reduced proliferation ( Fig. 6e ). The latter defect in combination with the increased liver/body weight ratio suggested hypertrophy of hepatocytes, and this was confirmed by analysis of cell size on staining of the actin cytoskeleton ( Supplementary Fig. 3A ). This is consistent with the enlargement of hepatocytes observed on long-term treatment with Itgb1 siRNA [21] . 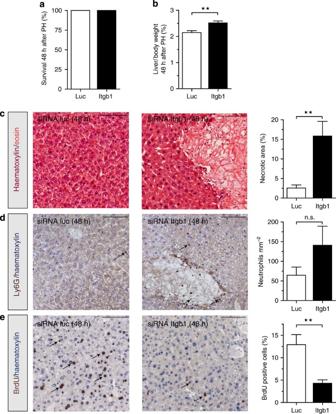Figure 6: Impaired liver regeneration in mice with Itgb1 knockdown. (a) Survival index 48 after PH.N≥12. (b) Liver-to-body-weight ratio 48 h after PH.N≥12. (c) Necrosis.N≥12. (d) Neutrophils.N≥5; Ly-6G-positive cells are indicated by arrows (e) BrdU-positive cells, 48 h after PH.N≥11. BrdU-positive nuclei are indicated by arrows. Scale bars, 100 μm (c–e). Bars represent mean±s.e.m. **P≤0.01 and ***P≤0.001 (Mann–WhitneyU-test). Figure 6: Impaired liver regeneration in mice with Itgb1 knockdown. ( a ) Survival index 48 after PH. N ≥12. ( b ) Liver-to-body-weight ratio 48 h after PH. N ≥12. ( c ) Necrosis. N ≥12. ( d ) Neutrophils. N ≥5; Ly-6G-positive cells are indicated by arrows ( e ) BrdU-positive cells, 48 h after PH. N ≥11. BrdU-positive nuclei are indicated by arrows. Scale bars, 100 μm ( c – e ). Bars represent mean±s.e.m. ** P ≤0.01 and *** P ≤0.001 (Mann–Whitney U -test). Full size image To test whether the liver necrosis that we observed after PH in mice with Itgb1 knockout or knockdown was due to enhanced sensitivity to the anaesthetic and/or analgesic compounds that we used during PH, we treated Itgb1 f/f /MxCre mice, Itgb1 knockdown mice and the corresponding control mice with isoflurane and buprenorphine, similar to the treatment used for PH. Forty eight hour later mice were killed, livers were analysed by haematoxylin and eosin staining and transaminase activities were measured in the serum. Importantly, neither knockout nor knockdown animals showed treatment-induced liver damage ( Supplementary Fig. 3B,C ). Transaminase activities of Itgb1 f/f /MxCre mice treated with isoflurane and buprenorphine were in the same range as in untreated Itgb1 f/f /MxCre mice ( Supplementary Fig. 1C ). Becuse of the better health status of the knockdown compared with the knockout mice and their survival post 48 h PH, we were able to analyse later stages of the regeneration process. Therefore, we next analysed the effect of Itgb1 knockdown 5 days after PH. The lasting knockdown at the 5-day time point was confirmed by quantitative reverse transcriptase–PCR (qRT–PCR) ( Fig. 7a ) and immunofluorescence staining ( Fig. 7b ). We also analysed an early time point (6 h after PH) and found no tissue damage in animals treated with siRNA either against luciferase or Itgb1 ( Fig. 7c ). Five days post PH, we still observed some necrotic tissue in the Itgb1 knockdown animals ( Fig. 7c ), but to a much lesser extent than 48 h post PH ( Fig. 6c ). Proliferation of hepatocytes had declined to almost basal levels in knockdown and control mice, and the liver-to-body-weight ratio was also similar at this late time point, demonstrating that regeneration can occur under these conditions ( Fig. 7d,e ). As we observed a uniform knockdown of Itgb1 even 5 days after PH, it seems unlikely to that cells with inefficient knockdown preferentially contributed to regeneration. Taken together, these data reveal that Itgb1 knockdown impairs liver regeneration, but does not prevent it. 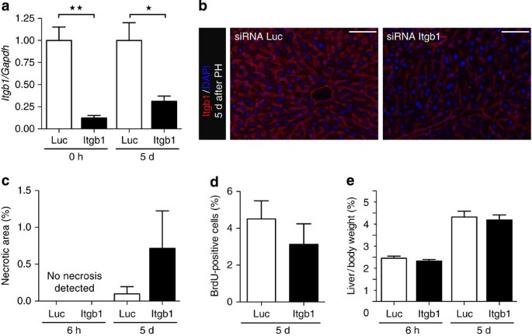Figure 7: Effect of siRNA-mediatedItgb1knockdown on liver regeneration 6 h and 5 days after PH. (a) Verification of siRNA-mediated knockdown ofItgb1mRNA by qRT–PCR (normalized toGapdh).N≥5 per treatment group and time point. (b) Immunostaining for Itgb1 (red) and DAPI nuclear counterstain (blue) on cryosections of tissue removed 5 days after PH. (c) Necrotic area 6 h and 5 days after PH.N≥5 per genotype and time point. (d) BrdU-positive cells 5 days after PH.N≥5. (e) Liver-to-body-weight ratio ofLucandItgb1siRNA-treated animals 6 h and 5 days after PH.N≥5. Scale bars, 100 μm (b). Bars inaandc–erepresent mean±s.e.m. *P≤0.05 and **P≤0.01 (Mann–WhitneyU-test). Figure 7: Effect of siRNA-mediated Itgb1 knockdown on liver regeneration 6 h and 5 days after PH. ( a ) Verification of siRNA-mediated knockdown of Itgb1 mRNA by qRT–PCR (normalized to Gapdh ). N ≥5 per treatment group and time point. ( b ) Immunostaining for Itgb1 (red) and DAPI nuclear counterstain (blue) on cryosections of tissue removed 5 days after PH. ( c ) Necrotic area 6 h and 5 days after PH. N ≥5 per genotype and time point. ( d ) BrdU-positive cells 5 days after PH. N ≥5. ( e ) Liver-to-body-weight ratio of Luc and Itgb1 siRNA-treated animals 6 h and 5 days after PH. N ≥5. Scale bars, 100 μm ( b ). Bars in a and c – e represent mean±s.e.m. * P ≤0.05 and ** P ≤0.01 (Mann–Whitney U -test). Full size image Itgb1 controls c-Met and EGFR activation As EGFR ligands and HGF are major mitogens for hepatocytes in the regenerating liver [1] , [3] and as mice lacking EGFR or the HGFR c-Met in the liver revealed similar regeneration abnormalities as the Itgb1 f/f /MxCre and Itgb1 knockdown mice [9] , [10] , [11] , we tested a possible involvement of impaired EGFR and/or c-Met signalling in the proliferation and survival defect of Itgb1-deficient hepatocytes. Levels of phosphorylated c-Met (Tyr1003) and EGFR (Tyr1068) were indeed reduced in Itgb1 knockout animals 0 and 48 h post PH ( Fig. 8a ), and reduced phosphorylation of EGFR was also observed in mice with Itgb1 knockdown 48 h after PH ( Fig. 8b ). Levels of total and phosphorylated focal adhesion kinase (FAK), a major relay of integrin signalling, were not affected by loss of Itgb1 ( Fig. 8a ). 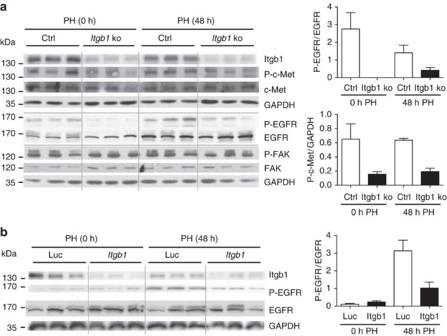Figure 8: Loss of Itgb1 affects phosphorylation of c-Met and EGFR during liver regeneration. (a) Immunoblotting of Itgb1, phosphorylated and total c-Met, EGFR and FAK, and of GAPDH (loading control) using homogenates from the livers of three poly-IC-treated control and Itgb1f/f/MxCre mice removed during surgery (0 h) and 48 h after PH. Densitometric analysis was performed for phosphorylated EGFR and c-Met. (b) Immunoblotting of Itgb1, phosphorylated and total EGFR and GAPDH using homogenates from the livers of threeLucorItgb1siRNA pre-treated animals removed during PH (0 h) and after 48 h. Densitometric analysis was performed for phosphorylated EGFR. Bars represent mean±s.e.m.N=3. Figure 8: Loss of Itgb1 affects phosphorylation of c-Met and EGFR during liver regeneration. ( a ) Immunoblotting of Itgb1, phosphorylated and total c-Met, EGFR and FAK, and of GAPDH (loading control) using homogenates from the livers of three poly-IC-treated control and Itgb1 f/f /MxCre mice removed during surgery (0 h) and 48 h after PH. Densitometric analysis was performed for phosphorylated EGFR and c-Met. ( b ) Immunoblotting of Itgb1, phosphorylated and total EGFR and GAPDH using homogenates from the livers of three Luc or Itgb1 siRNA pre-treated animals removed during PH (0 h) and after 48 h. Densitometric analysis was performed for phosphorylated EGFR. Bars represent mean±s.e.m. N =3. Full size image To test whether Itgb1 directly controls hepatic EGFR signalling, we injected EGF intraperitoneally (i.p.) into mice with Itgb1 knockout or knockdown and analysed EGFR activation. Fifteen minutes after EGF injection, we observed strong phosphorylation of the EGFR in control animals, but not in knockout animals ( Fig. 9a ). Itgb1 knockdown mice showed increased levels of phosphorylated EGFR in unstimulated conditions, which, however, only mildly increased on EGF injection ( Fig. 9b ). To determine whether the inhibition of EGFR and c-Met signalling on loss of Itgb1 is a cell autonomous effect, primary hepatocytes were cultured after siRNA-mediated knockdown in vivo . Efficient knockdown of Itgb1 in cultured hepatocytes was confirmed by immunostaining and western blotting ( Fig. 9c,d ). Interestingly, EGF-induced EGFR phosphorylation was also abolished in cultured hepatocytes with Itgb1 knockdown ( Fig. 9d ). In contrast to the in vivo situation, basal levels of pEGFR were not increased on Itgb1 knockdown in vitro , indicating that the enhanced levels in vivo result from cell types other than hepatocytes. Concomitant with the impaired receptor phosphorylation, EGF-induced phosphorylation of Erk was strongly reduced and phosphorylation of Akt was abolished in cultured Itgb1 knockdown hepatocytes ( Fig. 9d ). HGF-induced phosphorylation of c-Met and Erk1/2 activation were also impaired in Itgb1 knockdown hepatocytes ( Fig. 9e ). In addition, internalization of fluorophor-labelled EGF was significantly diminished ( Fig. 9f ). Taken together, these findings demonstrate that loss of Itgb1 impaired EGFR and c-Met phosphorylation, EGFR internalization and activation of mitogenic signalling pathways downstream of EGFR and c-Met in hepatocytes. These abnormalities in growth factor signalling provide a plausible explanation for the impaired hepatocyte proliferation in the Itgb1 knockdown and knockout mice. 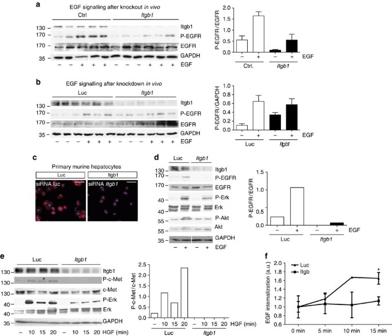Figure 9: Itgb1 controls growth factor receptor activation in hepatocytesin vitroandin vivo. Liver lysates from poly-IC-injected control and Itgb1f/f/MxCre mice (a), and from knockdown mice (b) 15 min after i.p. injection of EGF or vehicle were analysed by immunoblotting for Itgb1, phosphorylated and total EGFR and GAPDH (loading control). Densitometric analysis was performed for phosphorylated EGFR. Bars inaandbrepresent mean±s.e.m. (c) Itgb1 knockdown in primary hepatocytes prepared fromLucorItgb1siRNA pre-treated mice was confirmed by immunostaining for Itgb1 (red). Nuclei were countersained with DAPI (blue). Scale bars, 100 μm. (d,e) Primary hepatocytes were incubated for 15 min with EGF (d) or for the indicated periods with HGF (e). Lysates were used for immunoblotting of Itgb1, phosphorylated and total EGFR, c-Met, Erk, Akt and as loading control GAPDH. Densitometric analysis was performed for phosphorylated EGFR and c-Met. (f) EGFR internalization on stimulation with EGF was monitored by fluorescence-activated cell sorting analysis in primary hepatocytes fromLucorItgb1siRNA pre-treated mice.N≥3 per treatment group and time point. Values represent mean±s.e.m. *P≤0.05 (Mann–WhitneyU-test). Figure 9: Itgb1 controls growth factor receptor activation in hepatocytes in vitro and in vivo. Liver lysates from poly-IC-injected control and Itgb1 f/f /MxCre mice ( a ), and from knockdown mice ( b ) 15 min after i.p. injection of EGF or vehicle were analysed by immunoblotting for Itgb1, phosphorylated and total EGFR and GAPDH (loading control). Densitometric analysis was performed for phosphorylated EGFR. Bars in a and b represent mean±s.e.m. ( c ) Itgb1 knockdown in primary hepatocytes prepared from Luc or Itgb1 siRNA pre-treated mice was confirmed by immunostaining for Itgb1 (red). Nuclei were countersained with DAPI (blue). Scale bars, 100 μm. ( d , e ) Primary hepatocytes were incubated for 15 min with EGF ( d ) or for the indicated periods with HGF ( e ). Lysates were used for immunoblotting of Itgb1, phosphorylated and total EGFR, c-Met, Erk, Akt and as loading control GAPDH. Densitometric analysis was performed for phosphorylated EGFR and c-Met. ( f ) EGFR internalization on stimulation with EGF was monitored by fluorescence-activated cell sorting analysis in primary hepatocytes from Luc or Itgb1 siRNA pre-treated mice. N ≥3 per treatment group and time point. Values represent mean±s.e.m. * P ≤0.05 (Mann–Whitney U -test). Full size image In this study we demonstrate (i) that β1-integrins in hepatocytes are essential for liver regeneration, (ii) that they execute the regeneration-promoting function by cooperating with growth factor signalling and (iii) that siRNA-mediated knockdown is a potent strategy to study gene function in the regenerating liver in vivo . The generation of knockout mice guarantees a complete loss of a protein, but it is time and cost intensive, and permits to delete only a few genes in a mouse. Furthermore, many abnormalities in humans do not result from a complete loss of a gene, but rather from reduced levels of (a) protein(s). Therefore, a knockdown approach can sometimes reflect more closely the situation that occurs in human diseases. In this study we describe the first phenotypic comparison of a genetic knockout with siRNA-mediated knockdown in vivo in a tissue regeneration model within one species. The similar phenotypes that we observed in knockdown and knockout mice highlight the usefulness of the siRNA approach. The slightly milder phenotype of the knockdown animals prevented the lethality associated with the knockout and thus allowed us to extend mechanistic studies. We chose to deplete Itgb1, as there is as yet little information on the role of individual integrins in liver regeneration. This is surprising, given their high expression level on hepatocytes and the extensive matrix remodelling that occurs early after PH, which was suggested to promote the onset of hepatocyte proliferation [28] . However, the consequences of the loss of individual integrin subunits for liver regeneration had previously not been determined. Our results revealed that complete loss of Itgb1 in hepatocytes using the loxP/Cre approach still enabled liver homeostasis for a limited period of time, but was detrimental for liver regeneration as reflected by the strongly enhanced lethality observed between 24 and 48 h after PH in knockout mice. As the underlying mechanism, we identified severe liver necrosis and strongly impaired hepatocyte proliferation. This defect was recapitulated after Itgb1 knockdown, although without lethality. This difference is not surprising, as—in contrast to a knockout—a knockdown approach never leads to a complete loss of the expression of a gene. Thus, very low levels of Itgb1 in hepatocytes already prevent lethality. It is also possible that remnants of type I interferons induced by the poly-IC treatment represent a further challenge for the liver, resulting in more severe liver damage in Itgb1 knockout mice. Although neither the knockout nor the knockdown approach that we used resulted in specific deletion of Itgb1 in hepatocytes, several results obtained in this study strongly suggest that the loss of Itgb1 in these cells is responsible for the phenotype: (1) the liver was the only tissue where an efficient knockout and knockdown was achieved, (2) co-stainings of liver sections for Itgb1 and cell-type-specific markers revealed that hepatic endothelial cells, activated stellate cells/myofibroblasts and Kupffer cells retained Itgb1 expression in the knockout and knockdown mice, (3) loss of Itgb1 in haematopoietic cells did not affect liver regeneration and (4) the impairment in growth factor signalling in the absence of Itgb1 was observed in cultured primary hepatocytes, demonstrating that this is a cell autonomous effect. Finally, the data presented in the accompanying manuscript demonstrate that loss of Itgb1 in hepatoma cells alone is sufficient to inhibit liver tumorigenesis [21] . It is important to mention that the minor reduction in Itgb1 levels that we observed in other tissues/cells on Itgb1 knockout or knockdown is most likely not functionally relevant, as a >50% reduction of Itgb1 levels appears to be required to induce phenotypic abnormalities in vivo as demonstrated by the lack of abnormalities in mice with heterozygous Itgb1 deletion [27] . Integrins assemble a large number of signalling and adaptor proteins at the adhesion site, which transduce integrin signals to various subcellular compartments. ILK is a major adaptor that directly binds the β1-integrin tail and plays essential roles in integrin-mediated actin re-organization and growth factor signalling. Therefore, it was unexpected that our phenotype markedly differed from the abnormalities observed in mice lacking ILK in hepatocytes [8] . The only similarities were the enhanced liver/body weight ratio, which was, however, much more pronounced in the ILK-deficient mice. By contrast, hepatocyte-specific Ilk gene disruption in mice resulted in excessive rather than delayed/impaired regeneration through sustained hepatocyte proliferation and inappropriate termination of the PH-induced regeneration process. This resulted in severe liver enlargement [8] . Our data suggest that Itgb1 controls negative regulators, such as ILK, as well as positive regulators, and the latter seem to dominate during liver regeneration in our mouse models. The liver regeneration phenotype that we observed in Itgb1 knockdown and knockout mice is remarkably reminiscent of the abnormalities seen in mice lacking c-Met or EGFR in hepatocytes, suggesting that Itgb1 signalling is required for signalling by these receptors. This hypothesis is strongly supported by several results obtained in this study: (i) levels of phosphorylated EGFR and c-Met were reduced after knockout or knockdown of Itgb1 in hepatocytes in the regenerating liver, (ii) EGF-induced receptor phosphorylation was diminished after knockout or knockdown of Itgb1 in hepatocytes in vivo , (iii) EGF- and HGF-induced receptor phosphorylation and subsequent Erk1/2 and Akt activation were decreased in primary hepatocytes after Itgb1 knockdown and (iv) EGF internalization was reduced after Itgb1 knockdown in primary hepatocytes. Taken together, these data strongly suggest that loss of Itgb1 in hepatocytes impairs EGFR and c-Met activation on the cell surface and/or after internalization on endosomes, resulting in attenuated intracellular signalling. These results are consistent with previous in vitro findings that demonstrated the importance of integrins for EGFR activation and signalling, whereby the interaction can occur at various levels [29] , [30] . For example, it has been reported that integrin-mediated EGFR phosphorylation may occur in the absence of EGF [31] , and that Itgb1 knockdown affects EGFR signalling and subsequent cell proliferation in human lung cancer cells through impairment of EGFR turnover at the cell membrane [32] . However, an effect of integrins on ligand-induced phosphorylation of EGFR and the subsequent receptor internalization as shown in our study has not been demonstrated yet. Most importantly, loss of Itgb1 not only affected the EGFR, but also c-Met, a second key factor in liver regeneration. Therefore, our findings unravel a more general role of Itgb1 in the growth factor receptor signalling cross-talk in hepatocytes. The impaired EGFR and c-Met signalling provides an obvious explanation for the proliferation defect that we observed in Itgb1 knockout and knockdown mice. This hypothesis is further supported by the similar regeneration abnormalities of mice lacking EGFR or c-Met in the liver, which also suffered from delayed proliferation and enhanced necrosis, resulting in increased mortality after PH [9] , [10] , [11] . The extensive necrosis and apoptosis is most likely to be a consequence of the failure to restore the liver mass required for efficient detoxification of exogenous and endogenous compounds. In addition, the loss of the pro-survival activity of the Itgb1/EGFR/c-Met axis may further contribute to the phenotype as suggested by the reduced EGF-mediated activation of Akt in the absence of Itgb1. These results highlight the importance of the cross-talk between growth factor and integrin signalling, and suggest that proper activation of growth factor receptors is a major role of integrins in regenerating tissues. Animals Mouse maintenance and experiments had been approved by the local veterinary authorities (Kantonales Veterinäramt Zürich or District Government of Upper Bavaria). The animals were free of pathogens, including mouse hepatitis virus. Mice with floxed Itgb1 alleles [22] were mated with MxCre mice [23] , which allow activation of Cre recombinase on treatment with poly-IC. Single and double mutant mice were injected i.p. twice with poly-IC (250 mg/animal poly-IC, Amersham Biosciences, Piscataway, NJ) with a time interval of 2 days. After additional 14 days, mice were used for experiments. siRNA-mediated knockdown The following siRNAs were used: Itgb1 : sense 5′-AGAuGAGGuucAAuuuGAAdTsdT-3′, antisense 5′-UUcAAAUUGAACCUcAUCUdTsdT-3′; Control: sense 5′-cuuAcGcuGAGuAcuucGAdTsdT-3′, antisense 5′-UCGAAGuACUcAGCGuAAGdTsdT-3′. 2′-OMe-modified nucleotides are in lower case and phosphorothioate linkages are indicated by ‘s’. siRNAs were formulated in lipid nanoparticles (C12-200 lipoids) [19] . Seven-week-old C57BL/6 male mice received formulated siRNA directed against luciferase or Itgb1 (0.5 mg kg −1 ) via tail vein injection in a volume of 5 ml kg −1 body weight at day 1 and day 5. At day 10, the knockdown efficiency was determined in the liver tissue that was removed during PH (0 h time point). Generation of bone marrow chimeric mice Bone marrow chimeras were generated by injecting 6 × 10 6 bone marrow cells from Itgb1 f/f /MxCre mice into the tail vein of lethally irradiated (7.5 and 6 Gy with 4 h in-between) 8-week-old male C57BL/6 mice [33] . Three weeks later, Cre expression in the haematopoietic system was induced by two i.p. injections of 250 mg of poly-IC (GE Healthcare, Little Chalfont, Buckinghamshire, UK) with a time lag of 2 days. Partial hepatectomy Eight- to ten-week-old male mice, which received food and water ad libitum before surgery, were anaesthetized by inhalation of isoflurane (2%). PH was performed in the morning between 0800 and 1200 h. [34] Three liver lobes, including the previously emptied gall bladder, were removed. After surgery, mice were injected with buprenorphine for analgesia (Temgesic; Essex Chemie AG, Luzern, Switzerland; 0.1 mg kg −1 of body weight). They were euthanized by CO 2 inhalation, and the remaining liver was harvested at different time points after PH for further analysis. Histology and histomorphometry Liver samples were fixed in 4% paraformaldehyde (PFA) in PBS or in 95% ethanol/1% acetic acid, and embedded in paraffin. Sections (3.5 μm) were stained with haematoxylin/eosin and photographed (3–5 pictures per animal); the necrotic area was determined morphometrically. For the identification of cell size, unfixed cryosections (10 μm) were fixed in 4% PFA/PBS and permeabilized for 5 min in 0.1% Triton-X100 in PBS. Unspecific binding sites were then blocked with 3% BSA/PBS for 30 min at room temperature (RT). Rhodamine-coupled phalloidin (Life Technologies, Carlsbad, CA) was applied to stain the actin cytoskeleton and incubated overnight at 4 °C. Nuclei were counterstained with 4′,6-diamidino-2-phenylindole (DAPI). Sections were mounted with Mowiol. Identification of proliferating cells Proliferating cells were identified by 5-bromo-2′-deoxyuridine (BrdU) labelling [35] . For this purpose, BrdU (Sigma, Buchs, Switzerland; 250 μg g −1 body weight) was injected i.p. Two hours later, mice were killed and the collected liver tissue was fixed in acidic ethanol (95% ethanol, 1% acetic acid), embedded in paraffin and sectioned (3.5 μm). Detection of BrdU-positive cells was performed by immunohistochemistry using a peroxidase-coupled antibody against BrdU (1:30 diluted; Roche, Rotkreuz, Switzerland). BrdU-positive cells were counted in four independent microscopic fields ( × 200 magnification) per animal. Terminal dUTP nick-end labelling The In Situ Cell Death Detection Kit (Roche, Basel, Switzerland) was used for the detection of apoptotic cells. LacZ staining and activity assay Non-fixed cryo-sections were stained with LacZ for the detection of β-gal activity [22] . Frozen sections (10 μm) were thawed for 1 h at RT and fixed in 4% PFA in PBS for 5 min. After washing in 0.02% NP-40, 0.1 g l −1 sodium deoxycholate, 3.8 g l −1 EDTA, 4 mM MgCl 2 , 200 mM K 2 HPO 4 , pH 7.4, slides were incubated in 0.5 g l −1 X-gal, 10 mM K 3 Fe(CN) 6 , 10 mM K 4 Fe(CN) 6 , 0.4 g l −1 sodium deoxycholate, 0.08% NP-40, 3.8 g l −1 EDTA, 2 mM MgCl 2 , 100 mM K 2 HPO 4 , pH 7.4, at RT overnight before mounting in Mowiol. For detection of β-gal activity in platelets, lysates were incubated at 37 °C in assay buffer overnight and absorbance was monitored photometrically at 420 nm. Serum collection and analysis Mice were euthanized by CO 2 inhalation and blood was taken by heart punctuation. After coagulation, serum was harvested and snap-frozen. It was analysed using a Cobas Integra 400 Chemistry Analyzer (GMI, Ramsey, MN) and the corresponding reagents (Roche). Injection of EGF into mice Murine EGF (Peprotech, Rocky Hill, NJ; 0.05 mg kg −1 body weight in 0.1% BSA in isotonic saline) was injected i.p. into mice. Growth factor treatment of primary mouse hepatocytes Murine hepatocytes were isolated by the two-step collagenase perfusion method and cultured as described [36] . In brief, 8–10-week-old mice were killed by tail vein injection of pentobarbital (2.5 mg per 10 g body weight dissolved in isotonic saline containing 1,000 I.E. heparin per ml). The liver was perfused for 6 min via the vena cava with Hank’s balanced solution (without Ca 2+ and Mg 2+ ), while the aorta descendens was cut caudal to the liver. In the second step, the liver was perfused with 120 ml Hank’s balanced solution containing 50 mg collagenase. The liver was removed and liver cells were isolated by agitation and collected by centrifugation (200 g , 2.5 min). After a second centrifugation step, hepatocytes were enriched and purified by Percoll gradient purification and resuspended in RPMI 1640. Cells were plated in 2 ml RPMI 1640 medium in six-well dishes coated with collagen R (Serva, Heidelberg, Germany; 0.2 mg ml −1 ) at a density of 4 × 10 5 cells per well, and left to adhere for 3 h. The medium was changed to remove non-attached cells, and after 30 min 10 ng ml −1 murine EGF or HGF were added. Cells were lysed at different time points after growth factor addition and analysed by western blotting. EGF internalization After adherence of hepatocytes for 3 h, the medium was replaced by ice-cold medium containing 10 ng ml −1 fluorescein-conjugated EGF (Life Technologies) and incubated for 30 min to allow efficient ligand binding. Cells were washed with ice-cold PBS, prewarmed RPMI was added and plates were incubated at 37 °C for 5 min to adjust the temperature. Internalization was stopped at different time points by placing samples on ice and washing for 5 min with 0.2 M acetic acid, 500 mM NaCl, pH 2.8. Cells were then washed with ice-cold PBS, scraped off the dish, transferred into tubes in 1% PFA, 110 mM glucose, 50 mM sodium azide in PBS and fixed for 20 min. After centrifugation, they were resuspended in 2.5 mM EDTA, 0.1% BSA, 15 mM sodium azide in PBS and analysed by fluorescence-activated cell sorting using FloJo software (TreeStar Inc., Ashland, OR). Identification of neutrophils by immunohistochemistry Paraffin sections of tissue fixed with 95% ethanol/1% acetic acid were incubated for 30 min in 12% BSA in PBS/0.025% NP-40 to block unspecific binding sites. The primary antibody (anti-Ly6G; BD Pharmingen, Allschwil, Switzerland) was diluted 1:1,000 in blocking buffer and incubated overnight at 4 °C. Sections were stained using the ABC Vectastain Peroxidase Kit (Vector Laboratories, Burlingame, CA) according to the manufacturer’s protocol, counterstained with haematoxylin, rehydrated and mounted. Detection of Itgb1 by immunofluorescence Unfixed cryosections (10 μm) were dried 30 min at RT, fixed for 20 min at RT in 4% PFA/PBS, permeabilized for 5 min in 0.1% Triton-X100 in PBS and unspecific binding sites were blocked in 3% BSA/PBS for 30 min at RT. A rat monoclonal antibody against Itgb1 (Millipore, Zug, Switzerland) was applied and incubated overnight at 4 °C at a dilution of 1:400. Sections were incubated with Cy3-conjugated secondary antibody (Jackson ImmunoResearch Laboratories, West Grove, PA), 1:600 diluted in 3%BSA/PBS and DAPI (Life Technologies), to counterstain the nuclei, and mounted with Mowiol. Co-immunofluorescence staining of liver sections For co-immunofluorescence staining of Itgb1 and F4/80, unfixed cryosections (10 μm) were equilibrated at RT, fixed for 10 min in −20 °C cold acetone, dried on air and rehydrated with PBS. After blocking for 1 h with Dako blocking solution, primary antibodies were applied for 1 h with a rat monoclonal Itgb1 antibody labelled with DyLight647 (1:200 diluted) and F4/80 antibody (1:200 diluted; BM8, Biolegend, San Diego, CA, conjugated with Alexa488). Nuclei were counterstained with DAPI. Images were taken using a Zeiss LSM 700 laser scanning confocal microscope. For co-staining of Itgb1 with α-SMA or PECAM-1, unfixed cryosections (10 μm) were dried 30 min at RT, fixed for 5 min at 4 °C in methanol, permeabilized for 5 min on ice in 0.1% Triton-X100/PBS, washed once in PBS and unspecific binding sites were blocked in 0.7% fish gelatin, 3% BSA, donkey serum 1:20 in PBS for 2 h at RT. After washing in PBS, the primary antibodies anti-Itgb1 (1:400 diluted; Millipore) and anti-α-SMA-Cy3 (1:400 diluted; Sigma) or anti-PECAM-1 (1:200 diluted; Milipore) were applied overnight at 4 °C. After washing, anti-rat-Alexa 488 (1:200 diluted; Jackson), anti-hamster-Cy3 (1:300 diluted; Jackson) and DAPI were applied for 1 h at RT. After washing in PBS, the samples were mounted. Staining for cleaved caspase-3 Unfixed cryosections (10 μm) were dried 30 min at RT, fixed for 15 min at 4 °C in methanol, washed once in PBS and unspecific binding sites were blocked in 3% BSA/PBS. After washing in PBS, anti-cleaved caspase-3 antibody (1:100 diluted; Cell Signaling, Danvers, MA) was applied overnight at 4 °C. After washing in PBS, anti-rabbit-Cy3 antibody (1:500 diluted; Jackson) and DAPI were applied for 1 h at RT, followed by washing in PBS and mounting. RNA isolation and qRT–PCR analysis Total cellular RNA was isolated from liver tissue as described [37] , including a DNase digest (Promega, Dübendorf, Switzerland). Complementary DNA synthesis and qRT–PCR were carried out as described previously [34] . The following primers were used: Gapdh : 5′-TCG TGG ATC TGA CGT GCC GCC TG-3′ and 5′-CAC CAC CCT GTT GCT GTA GCC GTA T-3′; Itgb1 5′-ATG CCA AAT CTT GCG GAG AAT-3 and 5′-TTT GCT GCG ATT GGT GAC ATT-3′. Preparation of protein lysates and western blot analysis Frozen tissue was homogenized in T-PER tissue protein extraction reagent (Pierce, Rockford, IL) containing Complete Protease Inhibitor Cocktail and PhosSTOP Phosphatase Inhibitor Cocktail (Roche). Lysates were cleared by sonication and centrifugation (13,000 r.p.m., 30 min, 4 °C), snap-frozen and stored at −80 °C. The protein concentration was determined using the BCA Protein assay (Pierce). Proteins were separated by SDS–PAGE and transferred onto nitrocellulose membranes. The following antibodies were used: anti-P-ERK1/2 (1:1,000 diluted), anti-P-Akt (S473; 1:1,000 diluted), anti-total Akt (1:1,000 diluted), anti-P-EGFR (Tyr1068; 1:1,000 diluted), (all from Cell Signaling), anti-total ERK1/2 (1:1,000 diluted), anti-P-FAK (Tyr379; 1:1,000 diluted; Life Technologies), anti-total FAK (1:1,000 diluted; BD Biosciences, San Jose, CA), anti-Itgb1 (1:400 diluted; Millipore), anti-P-c-Met (1:500 diluted; Sigma), anti-GAPDH (1:10,000 diluted;HyTest, Turku, Finland), anti-total EGFR (1:200 diluted), anti-total ERK1/2 (1:500 diluted), anti-total-c-Met (Tyr 1003; 1:500 diluted; all from Santa Cruz, Santa Cruz, CA) and anti-ASGPR2 (1: 1,000 diluted; Abcam, Cambridge UK). Uncropped scans of the most important western blottings are shown in Supplementary Fig. 4 . Statistical analysis Statistical analysis was performed using the Prism4 software (GraphPad Software Inc., San Diego, CA). Quantitative data are expressed as mean±s.e.m. Significance was calculated with the Mann–Whitney U- test; * P ≤0.05, ** P ≤0.01 and *** P ≤0.001. How to cite this article: Speicher, T. et al. Knockdown and knockout of β1-integrin in hepatocytes impairs liver regeneration through inhibition of growth factor signalling. Nat. Commun. 5:3862 doi: 10.1038/ncomms4862 (2014).